Mechanical adaptability of the Bouligand-type structure in natural dermal armour Arapaima gigas, a fresh water fish found in the Amazon Basin, resist predation by piranhas through the strength and toughness of their scales, which act as natural dermal armour. Arapaima scales consist of a hard, mineralized outer shell surrounding a more ductile core. This core region is composed of aligned mineralized collagen fibrils arranged in distinct lamellae. Here we show how the Bouligand-type (twisted plywood) arrangement of collagen fibril lamellae has a key role in developing their unique protective properties, by using in situ synchrotron small-angle X-ray scattering during mechanical tensile tests to observe deformation mechanisms in the fibrils. Specifically, the Bouligand-type structure allows the lamellae to reorient in response to the loading environment; remarkably, most lamellae reorient towards the tensile axis and deform in tension through stretching/sliding mechanisms, whereas other lamellae sympathetically rotate away from the tensile axis and compress, thereby enhancing the scale’s ductility and toughness to prevent fracture. Most hard biological materials, such as bone, antler and teeth, derive their structural integrity from their hierarchical architecture, as specific mechanical properties, such as strength, ductility and toughness, are developed at distinct structural features existing at different dimensions ranging from the nano- to millimetre length-scales [1] , [2] . Such hierarchical assembly allows a damage-tolerant (that is, strong and tough) material to be created from the basic building blocks of ductile, but soft, collagen molecules and stiff, but brittle, mineral nanocrystals: strength comes primarily from the ability of absorbing energy at small length-scales through composite deformation of the mineral and protein phases, whereas toughness primarily originates from larger length-scales that are able to influence crack growth [3] . Indeed, varying the assembly can create materials with vastly different macroscale mechanical properties suited for different load-bearing functions [4] . These biological materials are clearly nanoscale collagen–mineral composites; however, it is the organization of these features at higher structural levels that provides the means to develop specific mechanical properties for particular functions. The protective scales of the Arapaima fish ( Fig. 1a ) are a prime example of a biological material’s evolution for a particular function, there to specifically resist the bite of piranhas through multiple levels of defence provided by the scale’s hierarchical architecture. First, the scales’ aspect ratio (that is, length/thickness) and degree of imbrication (that is, exposed length/total length) ( Fig. 1b ) both not only provide flexibility during movement but also determine how much an individual scale will bend in response to a predatorial attack [5] . Second, scales commonly have graded material properties throughout their thickness [6] , [7] , [8] to resist both puncture and bending. For Arapaima gigas scales, there are two distinct macro-level regions ( Fig. 1c ): a hard, highly mineralized outer shell (~0.5 mm thick) and a collagen inner core region (~1 mm thick) [9] , [10] . The highly mineralized outer shell provides hardness to minimize local plasticity and promote tooth fracture at the point of penetration by the predator; however, it also reduces tensile or compressive stresses during flexure through its corrugated morphology, which limits how much of the scale is under high stress during bending [11] . As the scales will deform and bend in response to a predatory attack, the graded material properties through the scale thickness ensure that the larger deformations are in the inner core region, which can support greater amounts of plastic deformation than the hard but more brittle outer shell [7] . This inner core consists of collagen lamellae arranged in layers, some 50-μm thick, the lamellae being assembled from mineralized collagen fibrils ( Fig. 1c ), that is, twisted periodic arrays of collagen molecules, embedded with hydroxyapatite mineral nanocrystals ( Fig. 1e ). The uniqueness of the lamellar structure is that the fibril orientation is consistent within each lamella but the neighbouring lamellae are misaligned creating a so-called Bouligand-type or twisted plywood pattern ( Fig. 1 ) [9] , [10] , [12] . 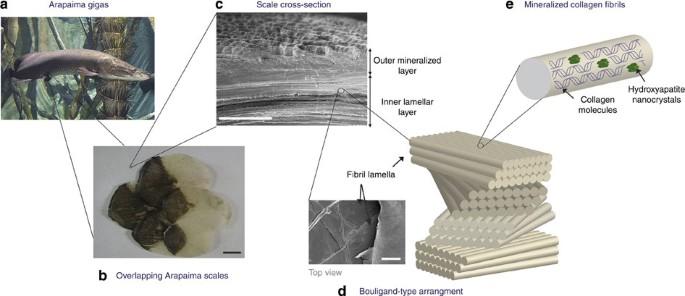Figure 1: Hierarchical structure of Arapaima gigas scales. (a) The scales of theA. gigasfish act as a natural dermal armour by providing multiple layers of defence. (b) First, the overlapping pattern allows flexibility through bending of multiple scales (scale bar, 20 mm). (c) TheArapaima gigasscale additionally has graded material properties through the cross-section consisting of a highly mineralized outer shell to provide hardness and an inner core of collagen fibril lamellae (scale bar, 0.5 mm). (d) The uniqueness of the Arapaima scales is that the lamellae are arranged in a Bouligand-type (or twisted plywood) pattern, such that the fibrils within neighbouring lamellae are rotated by various angles (scale bar, 200 μm). (e) Each lamella is composed of mineralized collagen fibrils with a predominantly parallel orientation. As in many biological materials, the fibrils ofA. gigasscales have two basic components: collagen and hydroxyapatite. The collagen molecules at the scale’s smallest length-scale form a staggered array with nanoplatelets of hydroxyapatite between the heads and tails of the collagen molecules. Adapted from Linet al.9 Figure 1: Hierarchical structure of Arapaima gigas scales. ( a ) The scales of the A. gigas fish act as a natural dermal armour by providing multiple layers of defence. ( b ) First, the overlapping pattern allows flexibility through bending of multiple scales (scale bar, 20 mm). ( c ) The Arapaima gigas scale additionally has graded material properties through the cross-section consisting of a highly mineralized outer shell to provide hardness and an inner core of collagen fibril lamellae (scale bar, 0.5 mm). ( d ) The uniqueness of the Arapaima scales is that the lamellae are arranged in a Bouligand-type (or twisted plywood) pattern, such that the fibrils within neighbouring lamellae are rotated by various angles (scale bar, 200 μm). ( e ) Each lamella is composed of mineralized collagen fibrils with a predominantly parallel orientation. As in many biological materials, the fibrils of A. gigas scales have two basic components: collagen and hydroxyapatite. The collagen molecules at the scale’s smallest length-scale form a staggered array with nanoplatelets of hydroxyapatite between the heads and tails of the collagen molecules. Adapted from Lin et al . [9] Full size image Here we investigate mechanical deformation in the novel assembly of mineralized collagen fibrils found in such ‘armoured’ Arapaima scales by using in situ synchrotron small-angle X-ray scattering (SAXS) during mechanical tensile tests to specifically analyse the deformation mechanisms originating from its Bouligand structure. We find that the Bouligand structure adapts to tensile loading by allowing the lamellar layers to rotate towards or away from the applied tensile stress, whereas thereby deforming in tension or compression, respectively. The lamellar layer’s ability to adapt to the loading environment is another mechanism within the scale contributing to the fracture resistance of this natural dermal armour. Diffraction from the Bouligand arrangement of lamellae When exposed to X-rays, the inner lamellar layer of the Arapaima scales creates a diffraction pattern that consists of distinct sets of concentric arcs, with each set appearing at a different angular orientation ( Fig. 2a ). These arcs result from the interaction of X-rays with the structure of the collagen fibril, which consists of a quarter-staggered array of collagen molecules with mineral nanoparticles within the gap regions situated between the heads and tails of the collagen molecules. The d -period of the alternating bands (that is, the distance between the centre of two gaps) measured here for the Arapaima scales was 64.6 nm (s.d. 0.3 nm). In the presence of X-rays, the entire fibril acts as a molecular diffraction grating due to the periodicity of the collagen–mineral composite structure, which has led to numerous studies on the structure and mechanical properties of collagenous tissues using X-ray diffraction [13] , [14] , [15] , [16] , [17] . 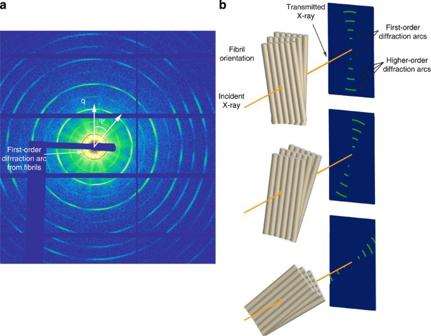Figure 2: Diffraction from Bouligand arrangement of lamellae. At the small-angle X-ray scattering (SAXS) beamline at the Advanced Light Source synchrotron, diffraction patterns from the inner layer of theA. gigasscales were collected. A representative diffraction pattern is shown ina. The periodicity in the mineralized collagen fibrils diffracts the incident X-rays at a small angle towards the detector. (b) The diffraction pattern generated by the fibrils creates concentric arcs parallel to the periodicity of the fibrils. In the Arapaima scale, the Bouligand-type arrangement of the lamellae diffracts the X-rays, such that distinct arcs may be observed at numerous orientations. Ina, the coordinates used to indicate direction in the diffraction patterns are given in terms of the radial direction,q, and the angle, ψ. Figure 2: Diffraction from Bouligand arrangement of lamellae. At the small-angle X-ray scattering (SAXS) beamline at the Advanced Light Source synchrotron, diffraction patterns from the inner layer of the A. gigas scales were collected. A representative diffraction pattern is shown in a . The periodicity in the mineralized collagen fibrils diffracts the incident X-rays at a small angle towards the detector. ( b ) The diffraction pattern generated by the fibrils creates concentric arcs parallel to the periodicity of the fibrils. In the Arapaima scale, the Bouligand-type arrangement of the lamellae diffracts the X-rays, such that distinct arcs may be observed at numerous orientations. In a , the coordinates used to indicate direction in the diffraction patterns are given in terms of the radial direction, q , and the angle, ψ. Full size image Figure 2a shows a representative small-angle X-ray diffraction pattern from an Arapaima scale in an unstressed state. In each set of concentric arcs, the arc closest to the beam centre—the first-order arc—corresponds to the d -period of the collagen fibril, whereas higher-order outer arcs correspond to harmonics of this period. The fact that concentric arcs appear at multiple distinct angles indicates that the scale has an architecture in which collagen fibrils exist in a number of specific orientations ( Fig. 2b ). Each set of concentric arcs corresponds to one distinct fibril orientation in the scale, with the angle of orientation in the fibril being given by the angle at the centre of the corresponding arc. Each arc has an azimuthal width and this width indicates a small distribution of fibril alignments around the central angle of orientation. The immediate visibility of a large number of higher-order arcs suggests that the level of mineralization in the inner layers of the scale is low. This conclusion is further supported by the small amount of diffuse scattering caused by mineral crystals and previous studies indicating a low mineral content [9] , [10] . On the basis of the fibrils being arranged in multiple distinct orientations, we conclude that the lamellae in the Arapaima scale have a Bouligand-type (twisted plywood) arrangement. We use the term Bouligand-type because a strict Bouligand structure may imply that the orientations occur at strictly uniform angular intervals. Our interpretation, however, is in agreement with a previous X-ray study that describes a similar architecture in the scales of the teleost fish Leuciscus cephalus [13] . Deformation within the Bouligand structure’s lamellae Using a high-flux synchrotron X-ray source, the orientations of the lamellae and the characteristic spacing of the collagen fibrils within each lamella can be measured in real time during a mechanical tensile test. When the scales are mechanically loaded, the change in the fibril’s arc position in q (its radial distance from the beam centre, in units of Å −1 ) indicates that the characteristic periodicity within the fibrils is either enlarging or contracting. Thus, a quantitative characterization of the local deformation in the collagen fibril lamellae can be performed simultaneously with the macroscopic deformation in the bulk sample. Similarly, by following changes in the azimuthal angle of the arcs, we can measure the changes in the orientation of each lamella. With the sample mechanically loaded in tension, diffraction patterns were collected in situ at regular intervals ( Fig. 3a ). A representative stress–strain curve is shown in Fig. 3b . Here, the stress and strain applied to the entire sample (that is, the tissue stress/strain) exhibit a linear curve up to 0.1 mm mm −1 strain, at which point the test was stopped. During mechanical testing, we found that the lamellae in Arapaima scales reorient in response to the loading. The reorientation is readily apparent just from observing the diffraction patterns; for example, a set of two-dimensional (2D) diffraction patterns from a representative test is shown in Fig. 3a , which were collected at the points indicated along the stress–strain curve ( Fig. 3b ). Before deformation begins (at point 1), one lamella is oriented at an angle ψ 0 =25.5° from the tensile axis and another at an angle ψ 0 =74°. With application of a tensile load to the sample, the arcs in Fig. 3a rotate; the arc closer to the tensile axis moves towards the tensile stress, whereas the arc at a greater angle moves away from it. 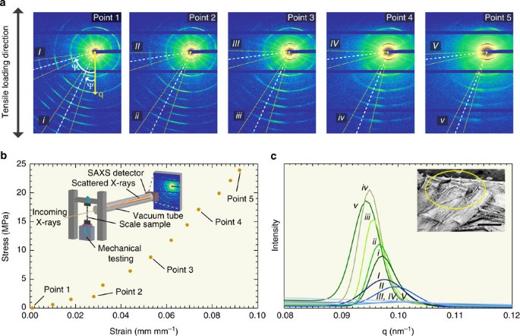Figure 3: Rotation and deformation inArapaima gigasscales. (a) The diffraction patterns are shown for five points during mechanical testing of a representative Arapaima scalein situduring small-angle X-ray diffraction measurements (see inset ofb). The corresponding stress–strain curve (that is, tissue stress versus tissue strain) is shown inb, which also marks the respective time points of the 2D diffraction images. At point 1 before testing, numerous fibril orientations are visible. Two fibril orientations are highlighted: one orientation is originally at an angle of ψ0~25.5° (i–v) to the tensile loading and the other is at roughly 74° (I–V), with a white dotted line denoting the centre of the arc and yellow lines tracing the general limits of the arc. As the load is applied to the sample, the orientation, ψ, of the arcs changes; in all figures, the white and yellow lines follow the centre of the moving arc. Here, we see that the fibrils closely oriented to the tensile axis reorient towards the tensile axis (i–v), whereas those at a larger angle move away from the tensile axis (I–V). (c) The 2D diffraction patterns were converted to 1D intensity versusqby integrating the intensity along the arc length for arcs (i-v) and (I–V) in the diffraction pattern for the first-order diffraction peak. Clearly, for lamellae oriented towards the tensile stress (i–v), the peak position has a negative shift inqindicating tensile strain; additionally, the intensity increases fromitovindicating that the rotation aligns the fibrils to create a higher density. The opposite effect occurs for lamellae misoriented with the tensile axis (I–V); the peak position has a positive shift inqindicating compressive strain and the peak disappears at higher strains, which may indicate interfibrillar separation (see inset, scale bar, 500 μm). Figure 3: Rotation and deformation in Arapaima gigas scales. ( a ) The diffraction patterns are shown for five points during mechanical testing of a representative Arapaima scale in situ during small-angle X-ray diffraction measurements (see inset of b ). The corresponding stress–strain curve (that is, tissue stress versus tissue strain) is shown in b , which also marks the respective time points of the 2D diffraction images. At point 1 before testing, numerous fibril orientations are visible. Two fibril orientations are highlighted: one orientation is originally at an angle of ψ 0 ~25.5° ( i – v ) to the tensile loading and the other is at roughly 74° ( I – V ), with a white dotted line denoting the centre of the arc and yellow lines tracing the general limits of the arc. As the load is applied to the sample, the orientation, ψ, of the arcs changes; in all figures, the white and yellow lines follow the centre of the moving arc. Here, we see that the fibrils closely oriented to the tensile axis reorient towards the tensile axis ( i–v ), whereas those at a larger angle move away from the tensile axis ( I – V ). ( c ) The 2D diffraction patterns were converted to 1D intensity versus q by integrating the intensity along the arc length for arcs ( i-v ) and ( I – V ) in the diffraction pattern for the first-order diffraction peak. Clearly, for lamellae oriented towards the tensile stress ( i – v ), the peak position has a negative shift in q indicating tensile strain; additionally, the intensity increases from i to v indicating that the rotation aligns the fibrils to create a higher density. The opposite effect occurs for lamellae misoriented with the tensile axis ( I – V ); the peak position has a positive shift in q indicating compressive strain and the peak disappears at higher strains, which may indicate interfibrillar separation (see inset, scale bar, 500 μm). Full size image Figure 3c plots the intensity integrated over a sector as a function of q for the two highlighted sectors in Fig. 3a ; the one-dimensional (1D) peak closer to the tensile axis ( i-v ) rotates towards the tensile axis, becomes more intense and deforms in tension (that is, q value decreases), whereas the peak ( I–V ) further from the tensile axis rotates away, decreases in intensity and deforms in compression (that is, q value increases). Indeed, the fibrils clearly have numerous orientations before testing ( Fig. 3a , point 1) but as the mechanical test progresses, the intensity of the 1D peaks becomes brighter in the directions closer to the tensile axis because most lamellae rotate toward the tensile direction. The 1D peaks rotating away from the tensile direction become dimmer and in this case essentially disappear, which possibly indicates interfibrillar separation (see inset of Fig. 3c ). Besides the high intensity of collagen fibrils rotating towards the tensile axis, a closer examination of the peak orientations in all samples ( Fig. 4a ) indicates that when the original orientation of the lamellae, ψ 0 , is within 15–30° of the tensile axis, the lamellae reorient towards the tensile axis by an average of 6–8°. In contrast, those lamellae originally 61–90° from the tensile axis actually move away from tensile loading by an average of 6.75°. 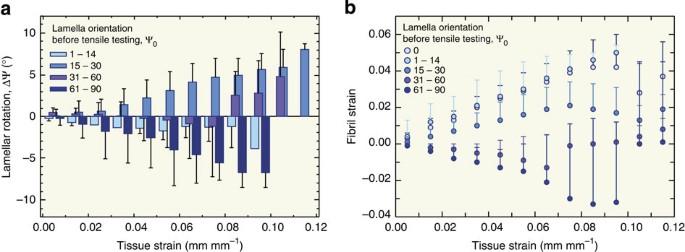Figure 4: Quantification of rotation and strain. As the scales are loaded in tension, the small-angle X-ray diffraction pattern indicates that the lamellae are rotating and deforming. Here, the (a) rotation and (b) strain in the fibrils is quantified as a function of the (macroscopic) tissue strain applied to the scale during the tensile test. Most significantly, our results indicate that lamellae originally oriented between 15–30° of the tensile axis rotate towards the tensile direction (+ rotation) and deform in tension, whereas those layers at an angle >60° rotate away from the tensile axis (− rotation) and deform in compression. The rotation and strain data derive from seven samples tested in tension, from which a total of 20 diffraction arcs were analysed: two arcs were between 1–14°, eight arcs were between 15–30°, five arcs were between 31–60° and five arcs were between 61–90°. Error bars represent the s.d. Figure 4: Quantification of rotation and strain. As the scales are loaded in tension, the small-angle X-ray diffraction pattern indicates that the lamellae are rotating and deforming. Here, the ( a ) rotation and ( b ) strain in the fibrils is quantified as a function of the (macroscopic) tissue strain applied to the scale during the tensile test. Most significantly, our results indicate that lamellae originally oriented between 15–30° of the tensile axis rotate towards the tensile direction (+ rotation) and deform in tension, whereas those layers at an angle >60° rotate away from the tensile axis (− rotation) and deform in compression. The rotation and strain data derive from seven samples tested in tension, from which a total of 20 diffraction arcs were analysed: two arcs were between 1–14°, eight arcs were between 15–30°, five arcs were between 31–60° and five arcs were between 61–90°. Error bars represent the s.d. Full size image As shown in Fig. 4b , the strain in the tensile direction and also in the reorienting fibrils was measured as a function of the strain applied to the whole sample. The lamellae originally oriented within 30° of the tensile axis rotate predominantly towards the tensile axis and stretch (deform in tension). In contrast, those lamellae originally oriented at higher angles to the tensile stress generally compress, while rotating away from the tensile axis. The dermal scales of the Arapaima fish are a prime example of how the structural arrangement of simple biological components can create armour with the capacity to be tough yet penetration resistant. The ability of the A. gigas ’ outer dermal layer to resist predatory attacks derives from its sophisticated structure from the nano- to macro-length-scales. The outer mineral layer gives the scale hardness and penetration resistance [9] , [10] , whereas the overlapping of the scales [5] and the corrugated outer surface of the mineral layer [11] allow the scales to bend transferring tensile stress to the inner lower-mineralized lamellae. Through our in situ small-angle X-ray diffraction measurements during mechanical tensile tests of the inner layer of Arapaima fish scales, we found that the unique structural Bouligand-type arrangement of the scale's inner collagen layer has the ability to stretch and reorient the collagen lamellae primarily towards the tensile stress, with some lamellae compressing and reorienting away from the tensile stress. These two effects observed in the SAXS measurements, namely, the changes in the angle ψ 0 of the collagen fibrils with the tensile axis and the stretching of the collagen fibrils, can be explained by four mechanisms, which are shown schematically in Fig. 5 : fibril rotation through interfibrillar shear, stretching of the collagen fibrils, tensile opening of interfibrillar gaps and ‘sympathetic’ lamella rotation. 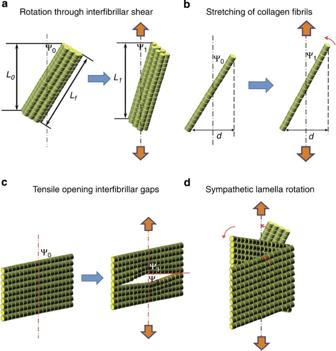Figure 5: Deformation and rotation mechanisms. The deformation and rotation phenomena in the scale’s Bouligand-type structure can be explained through four principal mechanisms. (a) Interfibrillar sliding causes rotation towards the tensile axis, where fibrils at an original orientation from the tensile axis of ψ0reorient to ψ1with a corresponding increase in projected length fromL0before loading toL1under loading with respect to the fibril length,Lf. (b) Elastic stretching of the lamellae could also cause the fibrils to rotate towards the tensile axis from ψ0to ψ1, whereas the projected length, (d), is assumed to remain unchanged. Other mechanisms within the Bouligand-type structure could be responsible for rotation away from the tensile axis. (c) Tensile separation of fibrils at an initial orientation of ψ0could force some fibrils to reorient toward the tensile axis (ψ2), whereas others rotate away from them (ψ1). Additionally, (d) ‘sympathetic’ rotation of lamellae could occur, where lamellae rotating towards the tensile axis force other lamellae to reorient away from the tension. Figure 5: Deformation and rotation mechanisms. The deformation and rotation phenomena in the scale’s Bouligand-type structure can be explained through four principal mechanisms. ( a ) Interfibrillar sliding causes rotation towards the tensile axis, where fibrils at an original orientation from the tensile axis of ψ 0 reorient to ψ 1 with a corresponding increase in projected length from L 0 before loading to L 1 under loading with respect to the fibril length, L f . ( b ) Elastic stretching of the lamellae could also cause the fibrils to rotate towards the tensile axis from ψ 0 to ψ 1 , whereas the projected length, ( d ), is assumed to remain unchanged. Other mechanisms within the Bouligand-type structure could be responsible for rotation away from the tensile axis. ( c ) Tensile separation of fibrils at an initial orientation of ψ 0 could force some fibrils to reorient toward the tensile axis (ψ 2 ), whereas others rotate away from them (ψ 1 ). Additionally, ( d ) ‘sympathetic’ rotation of lamellae could occur, where lamellae rotating towards the tensile axis force other lamellae to reorient away from the tension. Full size image Fibril rotation towards the tensile axis was observed in the SAXS experiments. A mechanism to explain such fibril rotation towards the tensile axis is interfibrillar shear. The fibrils are connected by hydrogen bonds that can break and reform by the shear component of the applied stress. Figure 5a shows how the relative sliding of the fibrils reorients them from ψ 0 to ψ 1 (ψ 1 <ψ 0 ). Gautieri et al . [18] modelled interfibrillar sliding in terms of the areal concentration of hydrogen bonds and obtained a force of 2.5 nN for a hydrated collagen molecule of length 20 nm. The strain ε can be expressed as ( L 1 – L 0 )/ L 0 ( Fig. 5a ), where the projected lengths L 1 (under loading) and L 0 (before loading) are determined through their relationship with the fibril length L f . As the deformation angle relates to the fibrillar length by cosψ 0 =( L 0 /2)/( L f /2) and cosψ 1 =( L 1 /2)/( L f /2), then the strain ε generated from collagen fibril rotation is cosψ 1 =( ε+ 1)cosψ 0 . Another mechanism that would result in rotation of the fibrils towards the tensile stress is stretching of the collagen fibrils. When the collagen fibrils are elastically stretched, they undergo a reorientation ( Fig. 5b ). To a first approximation, the lateral dimensions can be assumed unchanged. Here as sinψ 0 = d / L f and sinψ 1 = d / L f (1+ ε ), then sinψ 1 /sinψ 0 =1/(1+ ε ). Fibrils additionally were observed to rotate away from the tensile axis. One mechanism allowing this behaviour is tensile opening of interfibrillar gaps. If a lamella is highly misoriented with the tensile stress, the fibrils can separate by opening. One such event is shown in the scanning electron micrograph in the inset of Fig. 3c and schematically in Fig. 5c . This opening mechanism reorients the lower portion of the fibrils towards the tensile axis (ψ 2 ), whereas the others move away from them (ψ 1 ). A further mechanism allowing rotation away from the tensile stress is ‘sympathetic’ lamella rotation. The central lamella, sandwiched between two lamellae that reorient themselves toward the tensile axis, can be rotated away from it, with an increase in ψ, if the bonding between the lamellae is sufficiently high ( Fig. 5d ). From the above mechanisms, interfibrillar shear and fibrillar stretching both act to principally decrease ψ (that is, cause rotation towards the tensile axis); however, the opening of interfibrillar gaps and sympathetic rotation can also increase ψ (that is, cause rotation away from the tensile axis). The stretching and compression of collagen fibrils can be explained in a similar manner. The imposed tensile tractions stretch the collagen fibrils elastically if their orientation is close to the tensile axis (small ψ), whereas fibrils making large angles with the tensile axis (large ψ) are compressed due to the Poisson’s contraction of adjacent lamellae, which is a function of the anisotropy of strain in the Bouligand structure. In the inset of Fig. 3c , the lateral dimension of the sample decreased in the region adjacent to failure; this would generate shrinkage (negative strain) in the lamellae with large ψ. These reorientation/deformation mechanisms within the scale’s inner lamellar layer provide a means for the A. gigas to develop further defence against predators. Previous studies addressing the mechanical properties of the A. gigas structure have attributed its deformation resistance to the isotropy that the Bouligand structure creates [9] . However, the use of in situ small-angle X-ray scattering simultaneously with tensile testing allows us to track the orientation of the lamellae and their deformation during mechanical testing. Thus, not only does the Bouligand structure give a certain degree of isotropy to the mechanical properties, but the lamellae can also adapt to the loading conditions. Indeed, even though the actual loading conditions during a predatory attack include complicated stress-states, such as biaxial bending within the entire scale [5] or indentation/puncture [8] , [11] , the simple tensile tests implemented here demonstrate the possible contributions of the Arapaima’s Bouligand-type arrangement of lamellae towards deformation resistance. In summary, we have found a unique feature of the complex architecture and assembly of ‘armoured’ A. gigas fish scales, specifically that the Bouligand-type arrangement of the inner collagen fibril lamellae, with its originally isotropic structure, can adapt to loads in different orientations by reorienting the lamellae in response to stress. Using mechanical testing coupled with in situ SAXS, we have observed the lamellae rotating in response to loading; the majority of lamellae rotate towards the tensile stress and deform in tension, such that the fibrils stretch and slide along their principal orientation. In addition, some lamellae that are originally significantly misoriented with respect to the tensile stress direction (closer to 90°) rotate away from the tensile direction through mechanisms such as sympathetic rotation or interfibrillar opening and deform in compression due to the Poisson’s ratio effect. As the fibrils adapt to the loading environment, they increasingly contribute resistance to the bending of the full scale and thus enhance its fracture resistance. This enhanced flexibility of the lamellae, beneath the hard, but more brittle, penetration-resistant outer layer, provides protection to the sophisticated structure of A. gigas scales by increasing their ductility and toughness to resist their fracture. This represents a prime example of how natural materials have evolved their structure to generate desired multi-functionality, in this case to create dermal armour scales to resist external penetration without impairing flexibility. Sample preparation Seven rectangular samples were sectioned from A. gigas scales into 15 mm × 1 mm specimens. The samples were sectioned by holding the scale beneath a straight edge with two clamps and making straight, parallel cuts with a razor blade to achieve a reproducible geometry. The outer mineral layer was removed by polishing using sand paper from 180#–2,400#. The inner layer was also fine polished using sand paper from 1,200#–2,400# to achieve a flat sample with a thickness of roughly 0.6 mm. The scales were hydrated in water during the cutting and polishing procedures as well as for 12 h before mechanical testing. Mechanical testing with in situ small-angle X-ray scattering The hydrated Arapaima samples were loaded in tension, while exposing the samples to synchrotron X-rays at beamline 7.3.3 at the Advanced Light Source synchrotron radiation facility (Lawrence Berkeley National Laboratory, Berkeley, CA, USA). The mechanical tests were performed with a custom-made rig using a displacement stage and a 45-N load cell (Omega, LC703-10) to measure the force. The rig was such that SAXS data collection could be recorded in real time simultaneously with the measurement of the load–displacement curve. The mechanical tests were performed at room temperature and a displacement rate of 1 μm s −1 , with samples hydrated throughout the experiment by means of a hydration cell comprising a strip of cellophane held to the sample through capillary action with a few drops of water. A Pilatus 1M detector (Dectris Ltd., Baden, Switzerland) was used to collect the SAXS data. The detector was located at the largest allowable distance from the sample (~4,000 mm) to detect fine changes in the collagen peak’s position. The sample was exposed to X-rays for 0.5 s; data points were taken at ~5 s intervals. Tissue strain measurement The strain applied to the bulk sample was measured by marking the sample with four equally spaced horizontal lines: the full length between grips was 10 mm and the four lines were marked at roughly 2 and 4 mm from the centre of the span. A charge-coupled device camera was utilized to image the sample as the loads were applied. The macroscopic tissue strain in the sample was determined from the change in spacing of the outer horizontal lines on the sample during testing. The macroscopic tissue strain, ε t , applied to the samples can then be simply calculated as ε t =Δ l/l 0 , where Δ l = l i − l 0 is the change in length between the lines on the samples, and l i and l 0 are, respectively, their instantaneous and initial separations. Quantification of fibril orientation For each fibril orientation present, a sector with a width of 8° was centred on the peak in the 2D diffraction data and the angle, ψ, was recorded. The orientation of the fibril lamellae, ψ, with respect to the tensile axis was measured for each increment in tissue strain. After analysing the behaviour of the fibril lamellae, they were classified into groups based on the original orientation of the fibril before testing, which resulted in four groups: 1–14°, 15–30°, 31–60° and 61–90° from the tensile axis. For each sample, the fibril orientation values were binned for 0.01 increments in tissue strain; then, the binned values for each sample were averaged for each orientation group. From the seven samples tested in tension, a total of 20 diffraction arcs were analysed: two arcs were between 1–14°, eight arcs were between 15–30°, five arcs were between 31–60° and five arcs were between 61–90°. Quantification of SAXS fibril strain The fibril strain within the lamellae was measured by the change in the 1D peak position determined from the integrated intensity of the mineralized collagen fibril arcs. For the analysis, the software IGOR Pro (Wavemetrics) was used in conjunction with the custom macro NIKA (Jan Ilavsky, Argonne National Laboratory, Argonne, IL, USA) to calibrate the sample detector distance and beam centre with the 2D diffraction pattern of a silver behenate standard. This software was then used to convert the 2D SAXS data to 1D in the direction of the applied tensile stress as well as the other fibril lamella orientations present in each sample’s Bouligand structure. To convert the data to 1D, an 8° sector was positioned at a constant angle parallel to the tensile axis to obtain the fibril strain in the tensile direction by radially averaging the intensity over the sector. Because the fibril lamellae that are initially not parallel to the tensile stress are changing their orientation, the sector was positioned to follow the orientation of the moving peaks at each tissue strain increment. The 1D first-order and fifth-order mineralized collagen peaks were fit to an exponential Gaussian function and a linear background. The strain in the collagen fibrils was measured as the change in position of the first-order collagen peak’s centre divided by the strain at zero load. How to cite this article: Zimmermann, E. A. et al . Mechanical adaptability of the Bouligand-type structure in natural dermal armour. Nat. Commun. 4:2634 doi: 10.1038/ncomms3634 (2013).